Frequency-resolved optical gating capable of carrier-envelope phase determination Recent progress of the coherent light synthesis technology has brought the generation of single-cycle pulses within our reach. To exploit the full potential of such a single-cycle pulse in any applications, it is highly important to obtain the full information of its electric field. Here we propose a novel pulse characterization scheme, which enables us to determine not only the intensity and phase profiles of ultrashort pulses but also their absolute carrier-envelope phase values. The method is based on a combination of frequency-resolved optical gating and electro-optic sampling, which can be extended to a self-referencing scheme to determine the electric field evolution of few-cycle ultrashort pulses. We have experimentally demonstrated the technique to characterize sub-single-cycle infrared pulses, and numerically studied the capability of the scheme to incorporate a self-referencing technique and to extend the wavelength range to visible region. When one would like to measure an event in time, one usually has to use a reference event that is shorter than the event to be measured. Measurement of ultrashort light pulse duration (<10 −12 s) has been widely discussed for many years because no other shorter events are available as a reference. One of the most successful methods for the ultrashort pulse measurement is frequency-resolved optical gating (FROG) [1] , [2] , which is an innovative pulse characterization concept invented ~20 years ago. The concept is based on a spectrogram measurement, namely, recording a series of a nonlinear mixing signal between a pulse to be analysed (from here on called as test pulse) and a reference pulse by scanning the delay between the two pulses. This time-frequency method allows us to determine the intensity and phase evolution of an arbitrary ultrashort pulse without any assumption. One important feature is that the reference pulse does not need to be shorter than the test pulse, which means that self-referencing is possible with the scheme. This self-referencing capability is one of the largest advantages of the concept because it means that there is no limitation for measurable pulse duration. Another advantage is the versatility of applicable nonlinear interactions to mix the test and reference pulses. This allows us to apply the FROG concept for a very wide wavelength range. In fact, FROG has been applied from the mid-infrared [3] to extreme ultraviolet [4] regions so far. Further development of the ultrashort pulse-generation techniques enabled the generation of single-cycle pulses [5] , [6] , [7] , in which only one oscillation of the electric field exists. For such a pulse, its carrier-envelope phase (CEP), which determines the timing between the envelope and the carrier-wave, strongly affects the shape of the electric field. Consequently, full characterization of the electric field oscillating with a period of a few femtoseconds becomes significantly important. Unfortunately, FROG does not allow us to determine the CEP of the test pulse. One of the most famous methods to obtain full information of the electric field including the absolute value of the CEP is attosecond streaking [4] , [7] , [8] , [9] . In this method, both an extreme ultraviolet attosecond pulse and the test pulse are focused into a noble gas, and measurement of the kinetic energy of the photoelectrons produced by the extreme ultraviolet pulse reflects the vector potential induced by the test field because the photoelectron kinetic energy is modulated by the integration of the test electric field. However, there are serious restrictions on the measurable pulses. For example, the intensity of the test pulse must be high enough to generate extreme-ultraviolet attosecond pulses. Another problem of the scheme in terms of an electric field measurement is that the test field must be in a shape that can generate a single attosecond pulse. Therefore, the method is not really suitable for characterization of an arbitrarily shaped electric field. Such an attosecond pulse generation is not a common technology yet, and the number of groups that can properly handle attosecond pulses is limited. In addition, it is a time-consuming measurement because one has to measure photoelectrons ejected to a limited direction, and huge and expensive apparatuses are necessary to deal with attosecond pulses and high vacuum. Electro-optic sampling (EOS) [10] is another method to obtain a complete waveform of a few-cycle pulse. It is a very common technique to measure the field evolution of terahertz pulses. Typically both a terahertz pulse and a reference pulse are focused onto a nonlinear crystal, and the terahertz pulse induces a birefringence in the crystal through an electro-optic effect, which changes the polarization state of the reference pulse. The differential signal detected by using an ellipsometry technique [11] is proportional to the terahertz field at the time of overlap between the two pulses. By scanning the time delay between the two pulses, we can retrieve the variation of the terahertz electric field as a function of time. However, the method requires a reference pulse shorter than the period of the electric field to be characterized, which means that self-referencing is in principle not possible with the method and hence the applicability of the method is limited. The scheme has been used in a rather long wavelength region, specifically, from terahertz to mid-infrared region [12] , [13] , [14] . In this article, we explain a new method to characterize an arbitrary ultrashort pulse with the full information of its electric field. The scheme is based on a combination of EOS and FROG. The marriage of the two concepts perfectly compensates for their drawbacks with each other, and have given birth to a markedly new ultrashort pulse characterization method. The novel pulse characterization scheme is ideal for characterizing single-cycle pulses. We have succeeded in an experimental demonstration of the scheme, and the CEP control of a sub-single-cycle pulse have been clearly observed. We have also performed numerical simulations to show the capability of the scheme to incorporate a self-referencing technique and to extend the wavelength range to visible region. At first, we explain the theory of the characterization scheme, starting with the extension of the EOS concept and following with the possibility to connect it to FROG. Later, experimental demonstrations of the waveform characterization of sub-single-cycle infrared pulses in scanning and single-shot operations are shown. At last, we show the numerical simulation results for waveform characterization of few-cycle 800 nm pulses with self-referencing, and discuss the possibility of self-referencing and extension of the wavelength range of the scheme. Theoretical description EOS is based on an electro-optic interaction that is commonly understood as a nonlinear interaction between a terahertz wave and an optical wave. The terahertz wave modulates the refractive index of a nonlinear crystal and changes the polarization of the optical wave passing through the crystal. This interaction can be also explained as interference between the optical wave and the sum or difference frequency of the terahertz and optical waves [15] . Here we assume that the terahertz wave is a test pulse, E test ( t ), which is a pulse to be characterized, and the optical wave is a reference pulse, E ref ( t ). The time-averaged intensity of the delayed superposition of the fields of the reference pulse and the sum frequency between the reference and test pulses is written as where ‹› denotes time average and α is a constant proportional to the nonlinear susceptibility of the sum-frequency generation, which is assumed as an instantaneous process. τ is the delay between the reference and test pulses. The first term is independent of the delay time. The second term is the intensity cross-correlation signal between the test and reference pulses. If the second term is spectrally resolved, it yields a cross-correlation FROG signal (XFROG) [16] . The third term is the EOS signal, in other words, the interference between a local oscillator field ( E ref ( t − τ )) and a nonlinear field ( E ref ( t − τ ) E test ( t )). Only this term is measured with the conventional EOS technique. If it is possible to assume as a delta function, which is usually the case for terahertz wave measurement, becomes , which provides the complete information of the electric field of the test pulse. Otherwise, the term gives the electric field convoluted with I ref ( t ). This means that the spectrum will be filtered with the Fourier transform of I ref ( t ). As a result, the EOS signal will be restricted to near-zero frequency region and therefore provides phase information only around that spectral region, where some oscillating signal is detected. For example, if we use a 10 fs gaussian pulse as the reference, the cutoff wavelength, or the shortest detectable wavelength, would be ~1.9 μm, where the signal decreases by four orders of magnitude. The essential point of the new scheme we present here is realization of the simultaneous measurement of the second and third terms of equation (1). Although the XFROG and EOS terms can be analysed separately to yield two individual phase terms, they should be identical because they show the phase information of the same pulse. As the EOS term provides the absolute phase information, we can also determine the absolute phase of the XFROG term by connecting the two phase terms, as long as there is a spectral overlap somewhere between the XFROG and EOS terms. This technique allows us to determine the absolute phase over the whole spectral region beyond the EOS detection limit (>1.9 μm at a 10-fs reference pulse) and thus to retrieve the electric field completely. The absolute value of the spectral phase will be preserved during the filtering as long as the Fourier transform of the reference pulse intensity is real, that is, the intensity is symmetric in time ( ). Although the scheme naturally requires the CEP stability during the measurement, single-shot measurements are in principle possible with the scheme. It should be noted that the pulse duration of the reference pulse can be much longer than that required for the conventional EOS technique. For example, the shortest measurable wavelength of the EOS technique is ~1.9 μm when a 10-fs gaussian reference pulse is used as discussed above. In contrast, the measurable wavelength range of our method is in principle determined only by the FROG signal, which means that the duration of the reference pulse does not affect the detectable wavelength range. As long as there is some spectral overlap between FROG and EOS signals, the relative spectral phase obtained with FROG can be corrected with the phase of the EOS signal. Another important point is that the scheme works with many variations of nonlinear mixing as is the case with FROG. When difference frequency generation is used as the nonlinear interaction, equation (1) can be rewritten by substituting E test ( t ) by , and we are to retrieve , which contains essentially the same information as E test ( t ). Even higher-order nonlinear interactions like four-wave sum or difference frequency generation can be used when we use the second harmonic (SH) of the reference field as the local oscillator field. The generalized equation can be written as where n is a positive integer. 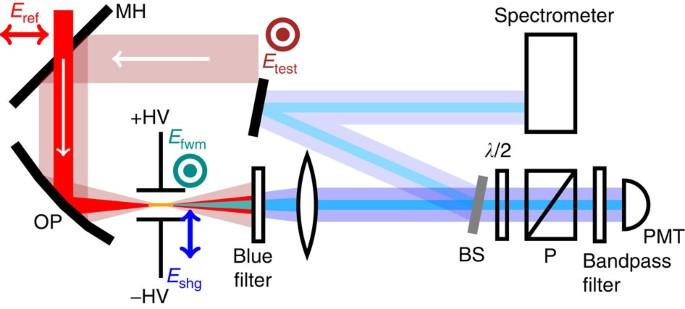Figure 1: Schematic of the system for scanning operation. BS, 7% beam splitter; HV, high voltage (4 kV); MH, mirror with a hole; OP, off-axis parabolic mirror; P, calcite polariser; PMT, photomultiplier tube. Table 1 summarizes how each term in equation (2) should be written when different nonlinear interactions are applied. It should be noted that polarization gating cannot be applied to our method because it is not possible to extract the phase information of the test pulse from the EOS term in this scheme. Table 1 The terms to be measured with cross-referencing. Full size table This flexibility also allows us to apply the concept for a very wide wavelength range as is the case with FROG. Although the theory is started from analysing the EOS signal for a terahertz wave, in the end there is no assumption in terms of the wavelengths of the input fields in the above discussion. Experimental demonstration An experimental demonstration of the scheme was realised with the system shown in Fig. 1 . The system is basically the same as the air-biased coherent detection scheme [17] , but the difference is that we simultaneously record the spectra of the signal at the same time. The detail of the system is described in the Methods section. The test pulse was a phase-stable sub-single-cycle infrared pulse ( E test ( t )) generated by using four-wave mixing through filamentation [18] . The reference pulse was a 30 fs 800 nm pulse ( E ref ( t − τ )) from a Ti:sapphire amplifier. The two beams were focused into nitrogen gas between high-voltage-biased electrodes and generated a four-wave difference frequency signal, , and the SH ( ) of the fundamental pulse at the same time and the same position. The intensity of the mixed fields is essentially obtained by using equation (2) as follows: Figure 1: Schematic of the system for scanning operation. BS, 7% beam splitter; HV, high voltage (4 kV); MH, mirror with a hole; OP, off-axis parabolic mirror; P, calcite polariser; PMT, photomultiplier tube. Full size image The beam generated through the nonlinear interaction was split into two; one beam was detected with a conventional spectrometer to obtain the spectrally resolved second term of equation (3), and the other beam was detected with a single-channel detector to obtain the third term of equation (3) by using an ellipsometry technique [11] . One important point of the experiment is that the SH and FWM signals should be generated at the same point to avoid an artificial phase shift between the two signals, which can affect the measured CEP value. One example of the data set is shown in Fig. 2a–c . 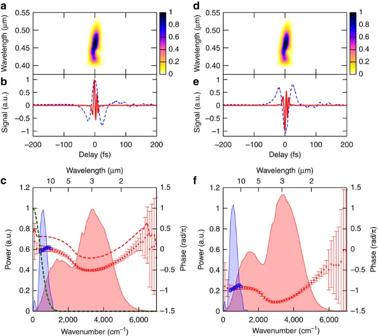Figure 2: Experimental results of the scanning operation. (a) The XFROG trace and (b) EOS signal (blue dashed curve) measured in the experiment. The red solid curve shows the electric field reconstructed with the method described in the text. (c) The red shaded and dashed curves are the spectral distribution and phase profile obtained with XFROG. The red dots are the spectral phase after the offset correction. The offset of the spectral phase is corrected by using the phase information obtained with EOS. The error bars of the phase are estimated with the bootstrap method described in the text. The blue shaded curve and open squares are the spectral distribution and spectral phase obtained from the Fourier transform of the EOS signal (dashed curve in (b)). The green dashed curve shows the filtering function for the EOS signal, which is Fourier transform of. The FROG error was 0.3% on a 512 × 512 grid. (d–f) are the experimental results where the CEP of the pulse changed by π from the pulse measured as the data set of (a) and (b). Figure 2a shows the measured trace of spectra corresponding to the second term in equation (3), and the dashed curve in Fig. 2b shows the measured signal corresponding to the third term in equation (3). The process of the field retrieval was as follows: (i) the intensity and (relative) phase of the test pulse in frequency-domain (the red shaded and dashed curves in Fig. 2c ) were obtained from Fig. 2a through an XFROG retrieval algorithm. The offset of the phase cannot be determined at this stage. (ii) The intensity and phase of the electric field in frequency-domain (the blue shaded curve and open squares in Fig. 2c ) was obtained through Fourier transform of the EOS signal (the dashed curve in Fig. 2b ). (iii) The spectral phase obtained with the XFROG was corrected by shifting it so that the spectral phases from XFROG and EOS match in the overlapped region, from 33 μm (300 cm −1 ) to 10 μm (1,000 cm −1 ), as the red closed circles in Fig. 2c ; (iv) the electric field of the generated infrared pulse with the corrected phase value was retrieved as the red solid curve in Fig. 2b . The full width at half maximum of the intensity in time-domain was 6.9 fs at 3.3 μm centre wavelength. The absolute phase at 3.3 μm was obtained as −0.51π. The phase shift at ~5 μm (2,000 cm −1 ) is due to interference between two different parametric processes at the generation of the infrared pulse [18] . Figure 2: Experimental results of the scanning operation. ( a ) The XFROG trace and ( b ) EOS signal (blue dashed curve) measured in the experiment. The red solid curve shows the electric field reconstructed with the method described in the text. ( c ) The red shaded and dashed curves are the spectral distribution and phase profile obtained with XFROG. The red dots are the spectral phase after the offset correction. The offset of the spectral phase is corrected by using the phase information obtained with EOS. The error bars of the phase are estimated with the bootstrap method described in the text. The blue shaded curve and open squares are the spectral distribution and spectral phase obtained from the Fourier transform of the EOS signal (dashed curve in ( b )). The green dashed curve shows the filtering function for the EOS signal, which is Fourier transform of . The FROG error was 0.3% on a 512 × 512 grid. ( d – f ) are the experimental results where the CEP of the pulse changed by π from the pulse measured as the data set of ( a ) and ( b ). Full size image It can be seen that the spectra and electric fields obtained from the EOS signals are the results of filtering by the Fourier transform of (the green dashed curve in Fig. 2c ). We can assume that the filtering function does not affect the phase value because the reference pulse was nearly gaussian and symmetric in time. The details of the filtering function are provided in the Methods section. Note that the slopes of the phases in the overlapped region coincide within the error bars, which means that the group delays from the two independent measurements are matched with each other. This fact strongly supports the consistency of the data sets. The accuracy of the spectral phases in the overlapped region obtained from the FROG and the EOS signals directly affect the accuracy of the waveform characterization. The phase obtained from the EOS signal can be very precisely defined because the oscillation period of the signal is much longer than the precision of the delay stage. The statistical error of the phase value from the EOS signal estimated through several measurements was ~0.01π. Determining the error of the spectral phase obtained from FROG is not so straightforward because the relationship between the measured data and retrieved values is complex in FROG. Here we have obtained the error bars by using a bootstrap method [19] , which is a well-established statistical resampling tool for determining uncertainty and has already been applied for the estimation of error bars of phases obtained from FROG [20] , [21] . We have estimated the s.d. of the phase in the overlapped region as 0.06π (see Fig. 2c ); therefore, the accuracy of the CEP is estimated as ±0.07π. If we use EOS alone with the 30-fs reference pulses to characterize the waveform, the measurable wavelength would be limited down to ~6.7 μm (1,500 cm −1 ), which is clear from the filtering function shown in Fig. 2c . However, the XFROG information can dramatically extend the detection range. We have demonstrated the pulse characterization down to ~1.7 μm (6,000 cm −1 ). Here we demonstrate that the scheme indeed allows us to detect the change of the CEP. It is known that the intensity of the infrared pulse generated by four-wave mixing changes with a period of ~200 nm by changing the delay between the fundamental and the SH of the Ti:sapphire laser output pulses [18] . The situation is similar to terahertz generation with gas plasma [22] , [23] . According to the references, the CEP changes by π when the delay is changed by ~200 nm. We tuned the delay between the fundamental and the SH by 200 nm and measured the XFROG trace ( Fig. 2d ) and the EOS signal of the pulse ( Fig. 2e ), whose CEP was expected to be shifted by π. Figure 2e,f shows retrieved electric fields in time- and frequency domain, respectively. As is expected, the intensity of the retrieved field does not change, whereas the CEP changes by π. Single-shot capability Extending our waveform characterization scheme to a single-shot operation would enable full characterization of CEP-unlocked laser pulses and would benefit significantly broader scientific fields. In particular, it could be very interesting for characterizing the pulses from free electron laser systems, where it is difficult to obtain CEP-stable pulses. Here we show some experimental proofs towards the single-shot measurement with this method. An experimental demonstration of the scheme in the single-shot operation was realised with the system shown in Fig. 3 . Basically, we combined the single-shot FROG [1] , [24] and single-shot EOS [25] , [26] , [27] techniques. The main idea of the single-shot detection is mapping the delay between the test and reference pulses onto the transverse position on the plane where the nonlinear interaction occurs. The detail of the system is described in the Methods section. The test and reference pulses were basically the same as those used in the scanning operation. The pulse front of the reference pulse was tilted with a calcium fluoride (CaF 2 ) brewster prism. The test and reference pulses were cylindrically focused into nitrogen gas between high-voltage-biased electrodes and generated a four-wave difference frequency signal and the SH of the fundamental pulse as was the case with the scanning operation. The signal was split into two and introduced into an imaging spectrograph with some polarization control and some vertical displacement (see Methods section). We recorded two vertically displaced traces simultaneously, and the vertical axis and the horizontal axis of each trace represent the delay and the wavelength, respectively. The intensity of the both traces are basically explained by spectrally resolving equation (3). The difference between the two traces is only the sign of the third term of the equation, which is extracted by the ellipsometry technique explained in the Methods section. By taking the sum and the difference of the two traces, the second and third terms can be completely split. The idea is based on the balanced terahertz air-biased coherent detection [28] . The sum (after subtracting the delay-independent first term as a background) corresponds to an XFROG trace, the second term of equation (3), and the difference corresponds to a spectrally resolved EOS signal, the third term of equation (3). We obtained the EOS signal by integrating the spectrally resolved EOS signal along the wavelength. The recorded traces and the retrieved pulse are shown in Fig. 4 . The pulse duration was 7.5 fs, which is slightly longer than that in the previous experiment, owing to a different filament condition. 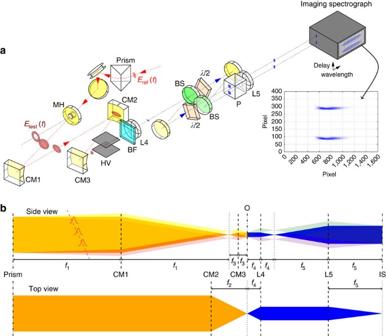Figure 3: Schematic of the system for single-shot operation. (a) System overview. BF, blue filter (FGB37, Thorlabs); BS, 50% beam splitter for 400–500 nm; CM1—3, concave cylindrical mirrors (f1=1000, mm,f2=190.7 mm andf3=51.9 mm, respectively); HV, high voltage (4 kV); L4,5, achromatic lenses (f4=75 mm, andf5=500 mm, respectively);λ/2, half-wave plate for 400–700 nm (newport); MH, mirror with a hole; P, calcite polariser; Prism, CaF2brewster prism. Inset shows a typical image recorded with the spectrograph. (b) Conceptual diagram of the imaging system. The red dashed line shows pulse front of the reference pulse tilted with the prism. Nonlinear interaction occurs at the point O. black dashed lines: positions of focusing optics, dotted lines: Fourier planes; IS, imaging spectrograph. The vertical image on the prism is transferred to the position O and the entrance of the imaging spectrograph. Figure 3: Schematic of the system for single-shot operation. ( a ) System overview. BF, blue filter (FGB37, Thorlabs); BS, 50% beam splitter for 400–500 nm; CM1—3, concave cylindrical mirrors ( f 1 =1000, mm, f 2 =190.7 mm and f 3 =51.9 mm, respectively); HV, high voltage (4 kV); L4,5, achromatic lenses ( f 4 =75 mm, and f 5 =500 mm, respectively); λ /2, half-wave plate for 400–700 nm (newport); MH, mirror with a hole; P, calcite polariser; Prism, CaF 2 brewster prism. Inset shows a typical image recorded with the spectrograph. ( b ) Conceptual diagram of the imaging system. The red dashed line shows pulse front of the reference pulse tilted with the prism. Nonlinear interaction occurs at the point O. black dashed lines: positions of focusing optics, dotted lines: Fourier planes; IS, imaging spectrograph. The vertical image on the prism is transferred to the position O and the entrance of the imaging spectrograph. 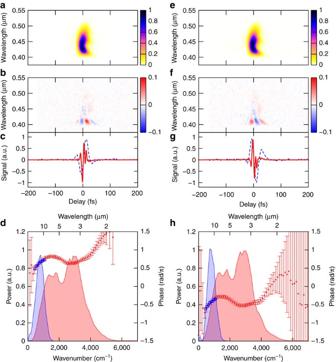Figure 4: Experimental results with the single-shot operation. Delay dependence of (a) sum and (b) difference of the two spectra described in the text. (c) The dashed curve was obtained by integrating the trace of (b) along the frequency axis. The solid curve shows electric fields reconstructed with the method described in the text. (d) The red shaded curve is spectral distribution with XFROG. The red closed circles are the spectral phase after the offset correction. The offset of the spectral phase is corrected by using the phase information obtained with EOS. The error bars of the phase are estimated with the bootstrap method. The blue shaded curve and open squares are the spectral distribution and spectral phase obtained from the Fourier transform of the EOS signal (dashed curve in (c)). The FROG error was 0.5% on a 512 × 512 grid. (e–h) are the experimental results where the CEP of the pulse changed by π from the pulse measured as the data set of (a) and (b). Full size image Figure 4: Experimental results with the single-shot operation. Delay dependence of ( a ) sum and ( b ) difference of the two spectra described in the text. ( c ) The dashed curve was obtained by integrating the trace of ( b ) along the frequency axis. The solid curve shows electric fields reconstructed with the method described in the text. ( d ) The red shaded curve is spectral distribution with XFROG. The red closed circles are the spectral phase after the offset correction. The offset of the spectral phase is corrected by using the phase information obtained with EOS. The error bars of the phase are estimated with the bootstrap method. The blue shaded curve and open squares are the spectral distribution and spectral phase obtained from the Fourier transform of the EOS signal (dashed curve in ( c )). The FROG error was 0.5% on a 512 × 512 grid. ( e – h ) are the experimental results where the CEP of the pulse changed by π from the pulse measured as the data set of ( a ) and ( b ). Full size image The exposure time of the camera was 2 s, corresponding to averaging 2,000 shots, to achieve a reasonable signal-to-noise ratio in the current condition. However, by optimizing the parameters such as the optical geometry and the gas for the nonlinear mixing [29] , [30] , [31] , [32] , we believe that it is possible to realize real single-shot detection with the concept. Self-referencing It is worth discussing the conditions for the self-referencing of the scheme because it is one of the most important features of pulse characterization schemes. As mentioned in the Introduction section, ultrashort light pulses are the shortest events that are available as a reference. As long as we cannot prepare and evaluate any events shorter than such light pulses, the only solution for the measurement of the ultrashort light pulses is to use themselves, namely, self-referencing. If this is possible, there is in principle no limitation for measurable pulse duration with the scheme. Although we used an independent pulse as a reference in our demonstration, self-referencing should be in principle possible because the electric field oscillation can be measured by using a reference pulse much longer than the period of the carrier-wave with the scheme. By substituting both E ref ( t ) and E test ( t ) by E ( t ), the equation (2) becomes Table 2 summarizes how each term in equation (4) should be written when different nonlinear interactions are applied in case of self-referencing. Second harmonic generation (SHG) can be applied if there is some overlap between the spectra of the fundamental and the SH. Third harmonic generation (THG) and self-diffraction can be applied if there is some spectral overlap between the SH (instead of the fundamental) and the generated signal. Polarization gating and transient-grating are not applicable because the phase information cannot be extracted from the mixed signal. From the above discussion, we can also conclude that the pulses that can be characterized with self-referencing must have a highly broadband, nearly one octave spectrum. Although this requirement sounds too demanding, it is rather reasonable because CEP values become important for few- or single-cycle pulses that have nearly one octave spectrum. Table 2 The terms to be measured with self-referencing. Full size table It is important to note that the phase of the filtering function affects the phase obtained from the EOS signal if the reference pulse is asymmetric. This could be a problem in case of self-referencing, where we cannot provide an independent reference pulse, and it is usually not trivial to perfectly remove the third-order dispersion (TOD) that makes the pulse asymmetric. However, it is possible to calculate the phase of the filtering function from the temporal intensity profile of the test pulse retrieved from the FROG signal. This information can be used to correct the phase modification caused by the pulse asymmetry. We performed a simple numerical simulation of the pulse characterization scheme with self-referencing. We assumed a 4.2-fs, phase-stable gaussian pulse at 800 nm with some TOD (the TOD of −20 fs 3 , the transform limit duration of 3 fs) as a test pulse. 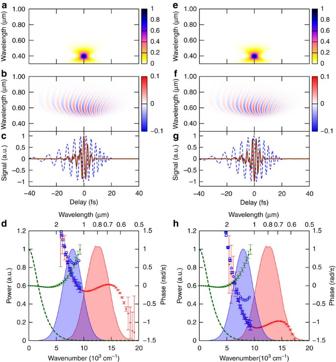Figure 5: Numerical simulations of the electric field measurement with self-referencing. The spectrally resolved (a) second term and (b) third term in equation (5). The test pulse is assumed as a 4.2-fs gaussian pulse at the carrier wavelength of 800 nm with some TOD (the TOD of −20 fs3, the transform limit duration of 3 fs). The phase of the test pulse at 800 nm is set to 0. (c) The dashed curve is obtained by intergrating the trace of (b) along the wavelength axis. The solid curve shows electric field reconstructed with the method described in the text. The test electric field (dashed green curve) is also shown. (d) The blue shaded curve and open circles are the spectral distribution and phase obtained from the Fourier transform of the EOS signal (dashed curve in (b)). The green dashed curve and closed circles show the amplitude and phase of the filtering function for the EOS signal, which is Fourier transform of |E(t)|2. The spectral phase of the EOS signal corrected with the phase of the filtering function (green closed circles) is shown as blue open squares. The red shaded curve and red closed circles are spectral distribution and phase, respectively, obtained with FROG shown in (a). The offset of the spectral phase is corrected by using the phase information of the EOS signal (blue open squares). The error bars are obtained with the bootstrap method described in the text. (e–h) are the simulation results where the phase of the target pulse at 800 nm is set to π. We simulated the SHG scheme of our pulse characterization method shown in Table 2 , namely, the following equation: Figure 5 shows the spectrally resolved second term, namely SHG-FROG trace, and the spectrally resolved third term. On the FROG trace, we have added random noise with the amplitude of 0.001 (relative to the peak). The same field retrieval as that shown in the main text was performed except for the phase correction by the filtering function. The filtering function was calculated by the Fourier transform of the temporal intensity profile obtained with the FROG signal. The phase of the filtering function (green closed circles in Fig. 5d,h ) was subtracted from the phase of the EOS signal (blue open circles in Fig. 5d,h ), and the phase (blue open squares in Fig. 5d,h ) was connected with the spectral phase obtained with the FROG signal. Figure 5: Numerical simulations of the electric field measurement with self-referencing. The spectrally resolved ( a ) second term and ( b ) third term in equation (5). The test pulse is assumed as a 4.2-fs gaussian pulse at the carrier wavelength of 800 nm with some TOD (the TOD of −20 fs 3 , the transform limit duration of 3 fs). The phase of the test pulse at 800 nm is set to 0. ( c ) The dashed curve is obtained by intergrating the trace of ( b ) along the wavelength axis. The solid curve shows electric field reconstructed with the method described in the text. The test electric field (dashed green curve) is also shown. ( d ) The blue shaded curve and open circles are the spectral distribution and phase obtained from the Fourier transform of the EOS signal (dashed curve in ( b )). The green dashed curve and closed circles show the amplitude and phase of the filtering function for the EOS signal, which is Fourier transform of | E ( t )| 2 . The spectral phase of the EOS signal corrected with the phase of the filtering function (green closed circles) is shown as blue open squares. The red shaded curve and red closed circles are spectral distribution and phase, respectively, obtained with FROG shown in ( a ). The offset of the spectral phase is corrected by using the phase information of the EOS signal (blue open squares). The error bars are obtained with the bootstrap method described in the text. ( e – h ) are the simulation results where the phase of the target pulse at 800 nm is set to π. Full size image The retrieval results are shown in Fig. 5c,g . As is expected, the test electric fields are well retrieved including the CEP information. The error bars of the phase, including the phase of the filtering function, are calculated with the bootstrap method as is the case with the experimental results. The accuracy of the CEP is estimated as 0.09π in this condition. Interestingly, time ambiguity does not exist in the scheme even if SHG-FROG is used. We also carried out a series of simulations by increasing the amount of the TOD while using the same spectrum as the previous simulation. The accuracy of the CEP decreases to 0.5π at the TOD of −75 fs 3 , where the pulse duration is 6 fs. Thus, the upper limit of the pulse duration can be estimated as 6 fs for characterization of 800 nm pulses with self-referencing. Waveform characterization methods reported so far can be classified into two categories: direct methods that measure the complete waveform and indirect methods that measure only the CEP and require additional phase profile measurements. Here we would like to discuss the difference between the two types of the waveform measurement methods. Using an f -to-2 f interferometer [33] , [34] together with a pulse characterization device such as FROG or SPIDER [35] , [36] would be a classical approach to obtain the information about both the pulse duration and the CEP of the test pulse at the same time. Although the f -to-2 f interferometer can detect the CEP drift even with single shot [37] , [38] , [39] , it is nearly impossible to obtain the absolute value of the CEP because there are many dispersive optical components that tremendously shift the CEP in the interferometer before the detection of the CEP signal. There are several methods with which we can clearly define the CEP value of the test pulse at a certain point. Typically in such methods, CEP values are estimated by measuring the CEP dependence of highly nonlinear signal and comparing the results with numerical simulations. For example, plasmonic sensors [40] , [41] , stereo-ATI (above-threshold-ionisation) [42] , [43] , [44] , [45] , velocity map imaging [46] , [47] , [48] , [49] and high harmonic generation [50] , [51] have been used for such purposes. With the help of a polarization gating technique, the CEP of multi-cycle pulses can be obtained [52] . However, to retrieve the complete waveform of the test pulse, the spectral phase must be obtained at a separate point from the CEP measurement. This requires extremely precise estimation of the dispersion difference between the two measurement points to achieve reasonable retrieval of the waveform of few-cycle pulses. Recently, it has been reported that the stereo-ATI signal alone is sufficient to estimate both the CEP and the duration of the pulses at the same time with the help of quantitative rescattering theory [53] , [54] , [55] or calibration with external SPIDER measurements [56] . However, the method is insensitive to the structures below 30% of the peak intensity. These methods indeed provide correct information about the main part of the pulses, which would be enough for high-field experiment. However, it does not give us the complete information of the waveform, which would be important for some other applications of few-cycle pulses such as high harmonic generation with a solid target. In our method, we measure the spectral phase and the CEP from different optical signals. However, there is no phase shift between these signals because the spectral phase and the CEP are measured at the same point. The waveform directly observed by using our method indeed reflects the waveform where the nonlinear mixing occurs, which is also the case for attosecond streaking and EOS. Among these methods, to our knowledge, our method alone has the capability to characterize the waveform of optical pulses with single-shot. In conclusion, we described and experimentally demonstrated a new concept to completely characterize the electric field of an ultrashort pulse, including the absolute value of the CEP. We have demonstrated the method by characterizing phase-stable sub-single-cycle 7 fs infrared pulses by using a 30 fs reference pulse, which is much longer than the period of the carrier-wavelength of the characterized pulse. We have also demonstrated that the method has the capability of single-shot measurements. The self-referencing possibility of the method has been also discussed with numerical simulations. The results of our numerical simulations have clearly shown that it is possible to retrieve few-cycle 800 nm pulses with the absolute CEP information by self-referencing. It has turned out that approximately one octave spectrum and reasonable compression quality are necessary for the self-referencing, which is rather reasonable requirement for the waveform characterization of few-cycle pulses whose CEP becomes important. In principle, the concept has no limitation to characterize few-cycle pulses on measurable pulse duration or applicable wavelength regions thanks to the self-referencing possibility. One example of interesting applications of the scheme is waveform characterization of the pulses delivered from a free electron laser. Currently, our method would be one of the best candidates to characterize the waveform of the optical pulses, whose spectrum and CEP changes shot-by-shot. Experimental setup for scanning operation An experimental demonstration of the scheme in the scanning operation was realised with the system shown in Fig. 1 . We generated phase-stable infrared sub-single-cycle pulses ( E test ( t ), 500 nJ, ω 0 ) by using four-wave mixing (FWM, ω 1 + ω 1 − ω 2 → ω 0 ) of the fundamental (700 μJ, 800 nm, ω 1 ) and the SH (15 μJ, 400 nm, ω 2 ) of Ti:sapphire amplifier (Femtopower compactPro, FEMTOLASERS) output through filamentation in nitrogen [18] . The centre wavelength of the generated infrared pulse was ~3.3 μm. The infrared pulse was combined with a small portion of the fundamental pulse ( E ref ( t − τ ), 15 μJ, 30 fs) with a delay time τ through a mirror with a hole. The combined beam was focused into nitrogen again with an aluminium-coated parabolic mirror ( f =150 mm). The polarizations of the reference pulse and the infrared pulse were perpendicular to each other, and the polarization of the generated FWM signal, , was parallel to the infrared pulse and perpendicular to the reference pulse. To produce SH ( ) of the reference pulse, a bias field was applied to Rogowski-type electrodes [57] with a distance of 3 mm by two high voltage amplifiers (HEOPS-5B6, Matsusada) with an amplitude of ±4 kV and a frequency of 500 Hz, which is synchronised with the 1-kHz repetition rate of the laser pulse train. The direction of the electric field was parallel to the reference pulse, and the FWM signal and the bias induced SH have polarizations perpendicular to each other. The beam generated through the nonlinear interactions was split by a beam splitter (sapphire plate) with nearly normal incidence. The reflected beam (~7%) was detected with a conventional spectrometer for XFROG. The transmitted beam was used for recording the EOS signal. The transmitted orthogonally polarized SH and FWM signals were mixed with a zero-order half-wave plate (WPH10M-405, Thorlabs) and the horizontally polarized component was selected through a calcite polariser. After passing through a bandpass filter at 400 nm (10 nm FWHM), the beam was detected with a photomultiplier tube (H10721-210, Hamamatsu). Interference between the SH and FWM signal was detected through a lock-in amplifier (SR830, Stanford Research) referenced with the modulation frequency of the high voltage (500 Hz). The interference signal does not affect the XFROG signal because the interference signal is much smaller than the FWM signal (<10% at 400 nm) and the integration time of the spectrometer (0.1 s) is much longer than the period of the modulation frequency of the high voltage. The required reference pulse energy for a reasonable signal-to-noise ratio was ~2 μJ with the current condition. Filtering and phase shift Here we describe the EOS signal with formulas to discuss the filtering effect and the phase shift in the EOS measurement at the current experimental setup. The bias-induced SH ( E shg ) and the FWM ( E fwm ) complex fields are given with slowly varying envelope approximation as where τ is the delay between the reference pulse and the test pulse, E bias is the bias field, and are the third-order nonlinear susceptibilities represented with the tensors [58] with the four subscripts corresponding to polarizations of the SH (or FWM), the bias field (or infrared), the fundamental and the fundamental beams, respectively. It is reasonable to approximate the third-order nonlinear susceptibilities to be constant and real because there is no absorption in nitrogen in the wavelength range from 400 nm to the infrared. These signals were mixed with a half-wave plate and one polarization component was selected with a polariser. The intensity of the selected component (horizontal polarization in this experiment), I ( τ ), is given as [11] where θ is the angle of the half wave plate. As the intensity of the SH signal is much weaker than that of the FWM signal, we only detect the heterodyne signal (the third term in equation (9)) with the lock-in amplifier. The signal becomes largest at θ =π/8. The detected signal becomes as follows by substituting equations (6) and (7), which is the full information of the test pulse field ( ) convoluted with . The Fourier transform of the signal is written as , where and are the Fourier transform of E test ( t ) and , respectively. The obtained power spectrum is written as , which is the spectrum filtered with the function of . The filtering function is also shown as a dashed curve in the Fig. 2c . It is clear that the high frequency cutoff of the spectrum at ~6.7 μm (1,500 cm −1 ) is due to the filtering effect. As C in equation (12) is real under our experimental condition, the only source that can make some additional phase shift is . When the intensity of the reference pulse is symmetric in time, namely, , is real and thus there is no additional phase due to this function. Our reference pulse satisfies such condition, which was confirmed with a FROG measurement. Experimental setup for single-shot operation An experimental demonstration of the scheme in the single-shot operation was realised with the system shown in Fig. 3 . The basic idea to realize the single-shot detection is to map the delay between the test and reference pulses onto transverse position on the plane where the nonlinear mixing occurs by tilting the pulse front of the reference pulse. Such a technology is common for single-shot FROG [1] , [24] and single-shot EOS [25] , [26] , [27] . The pulses used in the experiment were basically the same as those in the scanning experiment except for the pulse energies. The pulse energy of the reference (fundamental) pulse was increased up to 130 μJ to compensate for the reduction of the intensity where the nonlinear interaction occurred. On the other hand, the pulse energy of the test infrared pulse was reduced down to ~30 nJ to increase the contrast ratio of the FROG and EOS signals. The reference pulse with the beam size of 8 mm (1/ e 2 width) was sent through a calcium fluoride (CaF 2 ) brewster prism to tilt the pulse front of the beam. The calculated temporal range due to the pulse front tilt in this condition was ~450 fs. Not only the delay but also the dispersion experienced at each transverse position is different. We minimized the dispersion at the central part of the transverse position. The residual dispersion at each edge of the transverse position can be estimated as ±223 fs 2 , which introduces temporal broadening from 30 fs to 36 fs at each position. Such a situation is not ideal for precise pulse characterization but acceptable for the proof-of-principle experiment. The beam that passed through the prism was rotated by 90° with a periscope to have the pulse front tilt in the vertical direction. The infrared pulse was combined with the reference pulse through a mirror with a hole. To avoid undesirable spatio-temporal distortions due to the prism, the back surface of the prism was imaged by using a few cylindrical mirrors onto the plane where the nonlinear mixing occurred. The detail of the imaging geometry is shown in Fig. 3b . The precise imaging was confirmed by putting a mask very close to the prism and observing the image of the beam with a CCD camera. The beam was elliptical at the nonlinear interaction plane (O in Fig. 3b ), the vertical and horizontal 1/ e 2 widths being 400 μm and 50 μm, respectively. The polarizations of the reference pulse and the infrared pulse were perpendicular to each other, and the polarization of the generated FWM signal was parallel to the infrared pulse and perpendicular to the reference pulse. To produce the SH of the reference pulse, a DC bias field was applied to Rogowski-type electrodes [57] with a distance of 3 mm by two high-voltage amplifiers (HEOPS-5B6, Matsusada) with an amplitude of ±4 kV. The direction of the electric field was parallel to the reference pulse, and the FWM signal and the bias-induced SH have polarizations perpendicular to each other. The beam generated through the nonlinear interactions was split by a 1:1 broadband beam splitter (400–500 nm) with approximately normal incidence. The polarizations of the two beams were rotated by 45° and −45° respectively by using achromatic zero-order quartz-MgF 2 half-wave plates (10RP52-1, Newport) so that the two beams were cross-polarized to each other. The two beams were horizontally aligned but vertically displaced. The beams passed through a calcite polariser and only the horizontally polarized components transmitted. The transmitted beams were focused into an imaging spectrograph with an EMCCD camera (SP-2358 with ProEM+1600, Princeton Instruments). We were able to record two vertically displaced traces simultaneously. The vertical axis and the horizontal axis of each trace represent the delay and the wavelength, respectively. The signal of the two traces can be obtained by Fourier-transforming equation 8 after substituting θ =π/8 and θ =−π/8, respectively, as where denotes Fourier transform of E X ( t ) for each subscript. When the spectrum contributed from the delay-independent first term, , is subtracted as a background, the sum of the two spectra ( I SUM (ω, τ )) reflects the XFROG signal, and the difference between the two spectra ( I DIF (ω, τ )) reflects the EOS signal. These signals can be written as where is the Fourier transform of . When I DIF ( τ ,ω) is integrated along ω , we obtain where . This information is the same as equation (12). The exposure time of the camera was 2 s, corresponding to averaging 2,000 shots, to achieve a reasonable signal-to-noise ratio in the current condition. The required reference pulse energy for the measurement was ~80 μJ. The necessary reference pulse energy for the real single-shot measurement would be as high as ~3.6 mJ, which is estimated by simply multiplying 80 μJ by . However, such a parameter strongly depends on the experimental conditions such as the wavelengths of the pulses or kinds of nonlinear interactions. In addition, the development of highly sensitive and fast scientific CMOS cameras would be helpful to realize the real single-shot detection. How to cite this article: Nomura, Y. et al. Frequency-resolved optical gating capable of carrier-envelope phase determination. Nat. Commun. 4:2820 doi: 10.1038/ncomms3820 (2013).